Mapping ecologically relevant social behaviours by gene knockout in wild mice The laboratory mouse serves as an important model system for studying gene, brain and behavioural interactions. Powerful methods of gene targeting have helped to decipher gene-function associations in human diseases. Yet, the laboratory mouse, obtained after decades of human-driven artificial selection, inbreeding, and adaptation to captivity, is of limited use for the study of fitness-driven behavioural responses that characterize the ancestral wild house mouse. Here, we demonstrate that the backcrossing of wild mice with knockout mutant laboratory mice retrieves behavioural traits exhibited exclusively by the wild house mouse, thereby unmasking gene functions inaccessible in the domesticated mutant model. Furthermore, we show that domestication had a much greater impact on females than on males, erasing many behavioural traits of the ancestral wild female. Hence, compared with laboratory mice, wild-derived mutant mice constitute an improved model system to gain insights into neuronal mechanisms underlying normal and pathological sexually dimorphic social behaviours. With the sequencing of the mouse genome and the advent of large-scale mouse mutant production and of high-throughput phenotype analysis, the essential goal of obtaining a functional annotation of every gene in the mammalian genome is closer than ever. Achieving this goal will help decipher basic principles underlying mammalian biological processes in physiological and pathological conditions. Targeted gene mutation (knockout/knockin) in cultured embryonic stem cells derived from inbred laboratory mouse strains, usually in the 129/Sv genetic background and later backcrossed to C57BL/6 mice, is widely considered as the ‘gold standard’ approach to evaluate gene function in mammals and to provide preclinical models of diseases [1] , [2] . This strategy has already resulted in the production of thousands of mutant mouse models and numerous gene–phenotype associations [3] , [4] ( ftp://ftp.informatics.jax.org/pub/reports/ ). However, despite tremendous multidisciplinary efforts, the basic mechanisms underlying complex behaviours are still poorly understood, and the molecular and neuronal bases of social behaviours and their related disorders have remained elusive. It is well known that the phenotypes of mutant mice are largely influenced by the animal’s genetic background [5] , [6] , [7] . Virtually all classical laboratory mouse strains are derived from small founder populations and have been made genetically uniform (that is, homozygous for all genetic loci), hence facilitating experimental consistency and reproducibility. However, this artificial selection has resulted in a striking lack of genetic diversity in laboratory mouse models compared with natural animal populations, and has substantially reduced the genetic complexity of quantitative traits [8] , [9] , [10] , [11] , [12] . In addition, most laboratory mouse strains are the product of decades of artificial selection, both deliberate and inadvertent, that selected specific traits promoting reproductive success under laboratory conditions. For example, deliberate human selection interfered with locomotion, as well as with social and reproductive traits such as biting, aggressive conspecific competition, avoidance of mating with close relatives and fleeing/freezing predatory responses, that had evolved to maximize fitness in the natural environment [10] , [13] , [14] , [15] , [16] . Furthermore, captive mice in standard laboratory conditions are deprived of normal social context and lack social/reproductive pressures. As a result of decades of exposure to artificial and socially restricted environments, many behavioural traits with evolutionary adaptive purposes in nature have been inadvertently eroded. These multi-generational selections in ecologically irrelevant contexts have generated mouse strains with anatomical, physiological and pathological characteristics that are best adapted to domestic environments and that differ dramatically from those of the wild ancestors [17] . Thus, there is cause for concern about the validity of inbred laboratory mice as experimental models for studying ecologically relevant features that shape fitness in nature, as well as for identifying polygenic social traits and associated neuropsychiatric diseases [9] . In contrast, wild-derived mouse stocks provide a wide range of genetic variants and phenotypes, and offer the broad range of ecologically relevant traits of the Mus musculus that have disappeared in most classical laboratory mouse strains [18] . Wild-derived house mouse stocks differ in critical ways from wild-derived inbred laboratory strains or commercially available outbred laboratory strains: they are highly outbred; they contain marked genetic diversity and have undergone numerous recombination events between founder genomes, leading to higher mapping resolution [19] . Furthermore, wild-derived mice have been exposed for fewer generations to the artificial conditions of captivity, and are therefore likely to maintain behaviour alleles that are typically lost during the domestication process and the adaptation to vivarium conditions by standard laboratory strains [13] . Accordingly, we hypothesize that the investigation of gene mutations in the background of wild-derived mice should make valuable contributions to gene — phenotype associations studies unattainable in laboratory strains. In this study, we backcross a laboratory knockout mouse line with a laboratory knockout mouse line with wild-caught mice, thereby transferring the specific mutation from a standard inbred laboratory mouse strain onto an outbred wild-caught genetic background. Next, we perform a comprehensive phenotypic characterization of the morphology, physiology and behaviour of both male and female wild-caught mice, laboratory inbred mice and wild-backcrossed mice. We show that backcrossed mice display similar morphological, physiological and behavioural traits than those of wild-caught mice, including social and reproductive behaviours present in wild-caught females but absent in laboratory mice. Use of this novel mouse model enables us to study a rich resource of ecologically relevant behavioural traits that were profoundly altered or even lost in all classical laboratory (domesticated) mouse strains. Unexpectedly, we also observe a dramatic sex bias in phenotypic differences between the laboratory and the wild strains, suggesting that domestication preferentially affected or targeted the behavioural traits of females, and in particular social behavioural traits, while affecting to a much lesser extent the behavioural repertoire of males. To assess the applicability and potential of the wild-backcrossed mutant model system, we study here the function of the TrpC2 gene in female social and reproductive behaviours. Our results point to a novel role of this gene in wild-backcrossed females, in which female aggressive behaviour toward pups is activated by TrpC2 -mediated signals, a behavioural phenotype absent in the TrpC2 -mutant laboratory females. This finding indicates that gene mutations in recently derived wild mouse models provide a powerful approach to uncover neural mechanism underlying ecologically relevant behavioural traits that were lost or altered in the domestication process or under the artificial laboratory conditions or both. This strategy should yields novel insights into the basic mechanisms underlying social and reproductive responses and related human disorders. Generation of a wild-backcrossed knockout mouse model As a proof of concept of the applicability and scientific advantages of studying gene function on the genetic background of wild-derived house mice ( Mus musculus ), we backcrossed a commercially available inbred laboratory knockout mouse line with pathogen-free rederived wild mice (see Methods). Pathogen-free rederived wild mice were generated through the cross-fostering of newborn offspring from free-living wild-caught mice by post-partum CD-1 laboratory female mice [20] . We initiated a backcrossing breeding programme with eight rederived mice that were kept in captivity for seven generations. Wild-backcrossed mice were produced by 10-generation backcrossing of laboratory control TrpC2 +/− mice [21] with the rederived wild ( TrpC2 +/+ ) mice ( Fig. 1a ). To reduce inbreeding, each generation cross used individuals that were not the same as those used in the previous crosses and were neither the parents nor the siblings of any of the previously used mice. This backcrossing paradigm is expected to yield a mouse line with a genetic background consisting of >99% of the genetic background of the wild-caught mice, while incorporating the targeted gene mutation of the donor laboratory mouse strain. To determine the actual genetic makeup of the wild-backcrossed mice and determine the length of the flanking regions of the introduced TrpC2 -knockout locus of the laboratory strain in these mice, we compared the genotype of the entire chromosome 7 carrying the TrpC2 gene in 19 wild-backcrossed TrpC2 −/− mutant mice using the MegaMUGA high-density single-nucleotide polymorphism (SNP) array [22] , to that of the laboratory TrpC2 -mutant mice. The flanking region around the TrpC2 gene in the wild-backcrossed mutant mice was found to span approximately 8 Mbp (~0.3% of the total mouse genome), in agreement with the prediction for 10 backcrosses [23] (see Methods; Fig. 1b and Supplementary Data 1 ). 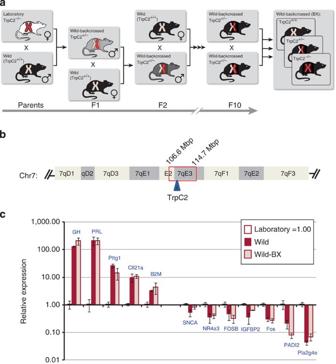Figure 1: Production and characterization of wild-backcrossed knockout mice, depicting restoration of traits lost or altered in domestication. (a) Backcrossing flowchart, describing the breeding procedure used to generate the F10 wild-backcrossed mutant mouse model targeting theTrpC2loci. (b) Schematic drawing of the position of the identified flanking region in the wild-backcrossedTrpC2-mutant mice. Flanking regions are marked in the red square box and the position of theTrpC2gene in the blue triangle. (c) Gene-expression profiling in the brains of wild-backcrossed mice is similar to that in wild mice. Relative expression of 12 genes, quantified from the hypothalamus of laboratory, wild and wild-backcrossed females using qPCR. The data show that the relative expression in the wild-backcrossed mice is similar to that of the wild mice and significantly different from that of the laboratory mice. Data are plotted as means±s.e.m.,n=3 mice per group (See alsoSupplementary Fig. 1). Figure 1: Production and characterization of wild-backcrossed knockout mice, depicting restoration of traits lost or altered in domestication. ( a ) Backcrossing flowchart, describing the breeding procedure used to generate the F10 wild-backcrossed mutant mouse model targeting the TrpC2 loci. ( b ) Schematic drawing of the position of the identified flanking region in the wild-backcrossed TrpC2 -mutant mice. Flanking regions are marked in the red square box and the position of the TrpC2 gene in the blue triangle. ( c ) Gene-expression profiling in the brains of wild-backcrossed mice is similar to that in wild mice. Relative expression of 12 genes, quantified from the hypothalamus of laboratory, wild and wild-backcrossed females using qPCR. The data show that the relative expression in the wild-backcrossed mice is similar to that of the wild mice and significantly different from that of the laboratory mice. Data are plotted as means±s.e.m., n =3 mice per group (See also Supplementary Fig. 1 ). Full size image Next, we examined whether the genomic similarity between the wild-backcrossed and the wild mice could also be observed in gene expression in the brain. To address this question we focused on gene expression in the hypothalamus, a region known to play a critical role in the regulation of social and reproductive behavioural and endocrine responses. We first performed genome-wide microarray expression analysis in the hypothalamus of female wild and laboratory mice (see Methods). Using code based on the R-package maskBAD, we checked the microarray data for possible differences in probe-binding affinity resulting from sequence differences between the laboratory strain and the wild strain. None of the probes showed significant differences in binding between strains (The false discovery rate, q >0.05 for all probes; see Supplementary Data 2 ). Surprisingly, we found significant differences in gene expression between wild and laboratory females (fold change >1.5 or <1.5, P <0.05) in 238 genes/predicted genes. Prominent among differentially expressed genes were genes that are reported to participate in the regulation of reproduction, social behaviours, and are associated with neuropsychiatric diseases, such as prolactin, growth hormone and the immediate early genes FOS and EGR1 ( Supplementary Fig. 1 ). To validate the identification of genes by microarray, we used quantitative PCR (qPCR) to assay the relative expression of 12 genes in the hypothalamus of wild and laboratory females. Genes identified by the microarray assays were selected for further validation on the basis of two criteria: a difference of >1.5-fold or <1.5-fold between the two strains ( P <0.05), and literature reports of involvement of the gene in the regulation of behaviours, and particularly social and reproductive behaviours. We found that the relative expression profiles of 11 of the 12 genes obtained by the qPCR analysis matched the array profiles ( Fig. 1c ). Lastly, to determine whether gene-expression profiles in the wild-backcrossed mice were similar to those in the wild mice, we used qPCR to analyse the relative expression levels of each of these genes in the same brain region of the two mouse strains. In all cases, we found that the gene-expression profiles in the wild-backcrossed females were similar to those in the wild mice and significantly different from those in the laboratory mice ( Fig. 1c ). Taken together, our analysis demonstrates that the genetic profiling of wild-backcrossed mice strongly resembles that of wild mice. Wild-backcrossed, laboratory and wild mice characterization Next we characterized the phenotypes of male and female laboratory TrpC2 +/+ control mice, wild-backcrossed TrpC2 +/+ control mice and wild house mice. All tested mice were raised and bred under the same laboratory conditions for several generations before the initial phenotypic testing. Our phenotypic assays consisted in a series of identically performed morphological, physiological and behavioural characterization. We hypothesized that the phenotype of wild-backcrossed mice was likely to be similar to that of their wild-caught counterparts and different from that of laboratory mice. In males, we found that compared with laboratory mice, both wild-backcrossed and wild mice were significantly smaller, weighed less and consumed less food and water. Wild-backcrossed and wild males also exhibited significantly higher anxiety/stress-related behaviours and about four times higher basal corticosterone levels than those of male laboratory mice (see Methods and Supplementary Table 1 ). There were no significant differences between the three mouse strains in locomotor (for example, velocity, distance travelled) or wildness-related behaviours (for example, spontaneous jumping and freezing). With regard to social behaviour, no significant difference was observed between the three mouse strains in aggressive behaviour toward intruder males or in pup-directed aggressive (infanticidal) behaviour ( Supplementary Table 1 ). Wild-backcrossed females, like males, exhibited morphological and physiological phenotypes similar to those of wild mice, and were significantly smaller, weighed less and consumed less food and water than laboratory mice ( Supplementary Table 1 ). In addition, locomotor and anxiety-related behaviours of wild-backcrossed and wild females were significantly more pronounced than those of laboratory females. For example, in the light/dark transition test (widely used to measure anxiety-like behaviours), the latency to first entrance into the light chamber was 2.2 s for laboratory females compared with more than 30 s for wild and wild-backcrossed females ( Fig. 2b and Supplementary Table 1 ). Corticosterone levels in both wild and wild-backcrossed females were also significantly higher than in laboratory females ( Fig. 2a ). In contrast to males, however, female mice displayed dramatic differences in all wildness-related behaviours and social behaviours. Wild-backcrossed and wild females exhibited high levels of wildness-related behaviours including spontaneous jumping and freezing behaviours, whereas no such behaviours were observed in laboratory females ( Supplementary Table 1 ). In the resident-intruder assay, wild-backcrossed and wild females spent significantly less time in olfactory investigation of a female intruder ( Fig. 2c ). Furthermore, wild-backcrossed females displayed a battery of social behaviours, such as pup-directed aggressive and female — female aggressive behaviour which, although typically robust in wild mice, are hardly ever seen in females of classical inbred laboratory strains ( Fig. 2d,e and Supplementary Table 1 ). 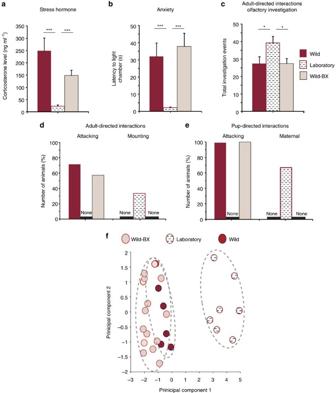Figure 2: Phenotypic characterization of wild-backcrossed (TrpC2+/+) females compared to wild females and laboratory (TrpC2+/+) females. (a) Serum corticosterone levels in wild, laboratory and F10 wild-backcrossed females. (b) Latency to entrance into the light chamber in the light/dark transition test for evaluating anxiety/stress-related behaviour. (c) Total olfactory investigation of adult female intruder. (d) Number of mice (%) exhibiting similar aggressive attacks (left) or mounting behaviour (right). (e) Number of mice (%) exhibiting pup-directed aggressive behaviour (left) or maternal behaviour (right). (f) Principal component analysis of 13 phenotypic traits of wild, laboratory, and wild-backcrossed females. Wild-backcrossed female mice are clustered together with wild female mice, and are statistically indistinguishable from them. All data are plotted as means±s.e.m., one-way analysis of variance followed by Fisher’s least significant differencepost hoctests; *P≤0.05, ***P≤0.005;n=7–18 mice per group. Figure 2: Phenotypic characterization of wild-backcrossed ( TrpC2 +/+ ) females compared to wild females and laboratory ( TrpC2 +/+ ) females. ( a ) Serum corticosterone levels in wild, laboratory and F10 wild-backcrossed females. ( b ) Latency to entrance into the light chamber in the light/dark transition test for evaluating anxiety/stress-related behaviour. ( c ) Total olfactory investigation of adult female intruder. ( d ) Number of mice (%) exhibiting similar aggressive attacks (left) or mounting behaviour (right). ( e ) Number of mice (%) exhibiting pup-directed aggressive behaviour (left) or maternal behaviour (right). ( f ) Principal component analysis of 13 phenotypic traits of wild, laboratory, and wild-backcrossed females. Wild-backcrossed female mice are clustered together with wild female mice, and are statistically indistinguishable from them. All data are plotted as means±s.e.m., one-way analysis of variance followed by Fisher’s least significant difference post hoc tests; * P ≤0.05, *** P ≤0.005; n =7–18 mice per group. Full size image Our behavioural phenotypic data are consistent with those reported by others, who concluded that the default in domesticated (inbred or outbred) mouse strains is calm behaviour, whereas the default in wild mice is anxious behaviour [24] , [25] . Furthermore, our data are compatible with studies showing that in wild mice, in contrast to domesticated mouse strains, both naïve males and naïve females present robust conspecific territorial aggression and infanticidal behaviour [26] , [27] . Overall, our wild-backcrossed mice demonstrated a robust set of behaviours that was qualitatively and quantitatively similar to that shown by wild mice ( Fig. 2f ). Lastly, comparison of phenotypic variability between the strains revealed, as expected, that in almost all behavioural measurements the variance within the wild-backcrossed mouse population was several fold higher than in the laboratory population but identical to that of wild mice. The greatest differences between the variance of the wild strains and the laboratory strain were found in the behavioural parameters, and specifically in the social and anxiety-related behavioural measurements in females ( Supplementary Table 1 ). Wild-backcrossed TrpC2 mutant females behaviour Social behaviours in mice are strongly regulated by pheromone signals, mediated largely by the vomeronasal system. To determine the usefulness of wild-backcrossed mice in defining the mechanisms underlying pheromone-evoked social behaviours, we generated wild-backcrossed mice harbouring a gene-targeted null mutation in TrpC2 . This gene is expressed in the vomeronasal organ and is essential for the detection of conspecific pheromone signals [21] , [28] , [29] . We then characterized sexually naïve (nulliparous) adult TrpC2 mutant and control females in a series of classical resident-intruder assays, using both wild-backcrossed and laboratory strains. We first assessed the role of TrpC2 in triggering territorial aggression in nulliparous females. The TrpC2 mutation produced no observable phenotypic change in female—female aggressive behaviour in the laboratory strain. In contrast, ablation of TrpC2 in nulliparous wild-backcrossed females led to significant repression of female-directed aggression, including reduction in the number of aggressive bouts and an increase in the latency to initiation of aggressive behaviour ( Fig. 3a,b ). Notably, the same mutation also produced an increase in the duration of olfactory investigation in both wild-backcrossed and laboratory females ( Fig. 3c ). 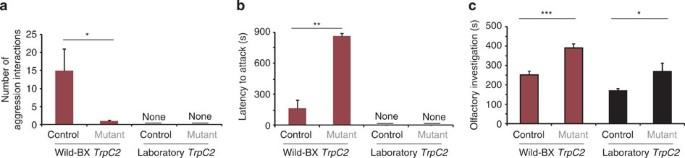Figure 3:TrpC2-mediated pheromone signals inducing female−female aggressive behaviour in wild-backcrossed mice. (a) Number of female–female attacks in controlTrpC2+/−and mutantTrpC2−/−mice, in laboratory and wild-backcrossed strains. (b) Latency to female-directed attacks. (c) Duration of olfactory investigation of an adult female intruder. Data are plotted as means±s.e.m., Student’st-tests; *P≤0.05, **P≤0.01, ***P≤0.005;n=10–12 mice per group. Figure 3: TrpC2 -mediated pheromone signals inducing female−female aggressive behaviour in wild-backcrossed mice. ( a ) Number of female–female attacks in control TrpC2 +/− and mutant TrpC2 −/− mice, in laboratory and wild-backcrossed strains. ( b ) Latency to female-directed attacks. ( c ) Duration of olfactory investigation of an adult female intruder. Data are plotted as means±s.e.m., Student’s t -tests; * P ≤0.05, ** P ≤0.01, *** P ≤0.005; n =10–12 mice per group. Full size image Next, we assessed the effect of TrpC2 -mediated pheromonal signals in the regulation of pup-directed behaviour in nulliparous females. Remarkably, 60% of the wild-backcrossed TrpC2 control females showed intense pup-directed aggressive behaviour and none exhibited nursing behaviour. In contrast, only 30% of the wild-backcrossed TrpC2 −/− mutant females showed pup-directed aggressive behaviour (and then only at moderate levels) and the rest of these females control either showed maternal behaviour or were indifferent to the newborn pups ( Fig. 4a ). Furthermore, the latency to initiation of pup-directed aggressive behaviour in the mutant wild-backcrossed females was almost double compared with the control wild-backcrossed females ( Fig. 4b ). In laboratory mice, in contrast, the TrpC2 mutation did not lead to any change in pup-directed aggressive behaviour ( Fig. 4a,b ). An increase in the initiation of maternal behaviour was observed in the mutant females in both the laboratory and the wild-backcrossed strains ( Fig. 4c ). 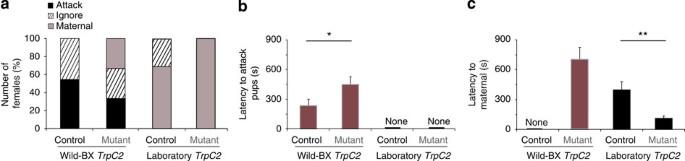Figure 4:TrpC2-mediated pheromone signals inducing pup-directed aggressive (infanticidal) behaviour in wild-backcrossed female mice. (a) Number of females (%) exhibiting maternal or pup-directed aggressive behavior toward alien newborn pups inTrpC2+/−andTrpC2−/−mice in the laboratory and wild-backcrossed strains. (b) Latency to pup-directed aggressive behaviour inTrpC2+/−andTrpC2−/−mice in the laboratory and wild-backcrossed strains. (c) Latency to maternal behaviour inTrpC2+/−andTrpC2−/−mice in the laboratory and wild- backcrossed strains. Data are plotted as means±s.e.m., Student’st-tests; *P≤0.05, **P≤0.01;n=10–12 mice per group. Figure 4: TrpC2 -mediated pheromone signals inducing pup-directed aggressive (infanticidal) behaviour in wild-backcrossed female mice. ( a ) Number of females (%) exhibiting maternal or pup-directed aggressive behavior toward alien newborn pups in TrpC2 +/ − and TrpC2 −/− mice in the laboratory and wild-backcrossed strains. ( b ) Latency to pup-directed aggressive behaviour in TrpC2 +/ − and TrpC2 − / − mice in the laboratory and wild-backcrossed strains. ( c ) Latency to maternal behaviour in TrpC2 +/ − and TrpC2 −/− mice in the laboratory and wild- backcrossed strains. Data are plotted as means±s.e.m., Student’s t -tests; * P ≤0.05, ** P ≤0.01; n =10–12 mice per group. Full size image Lastly, we found that wild-backcrossed and laboratory TrpC2 -mutant females demonstrated loss of olfactory sexual preference for approaching a male rather than a female ( Fig. 5b ). Furthermore, both wild-backcrossed and laboratory TrpC2 -mutant females exhibited heightened male-typical mounting behaviour toward intruder conspecific adult males as well as increased olfactory investigation toward an intruder mouse ( Fig. 5c–e ), consistent with previously reported findings in laboratory TrpC2 -mutant mice [28] . 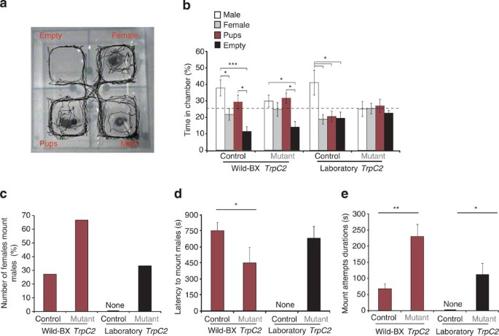Figure 5:TrpC2-mediated pheromone signals induce the loss of sexual olfactory preference and promote male-typical sexual behaviour. (a) Four-chamber social choice apparatus. Example of automated path tracking (curved line) of an experimental mouse, analysed with Ethovision software (Noldus). (b) Time spent (%) in each of the four chambers by laboratory and wild-backcrossed control and mutantTrpC2females. (c) Number of females presenting male-typical mounting behaviour toward an alien male mouse. (d) Latency to first male-typical mounting behaviour toward alien adult male mice by laboratory and wild-backcrossed control and mutant females. (e) Duration of male-typical mounting attempts toward an alien adult male. Data are plotted as means±s.e.m., one-way analysis of variance followed by Fisher’s least significant differencepost hoctest (b) or Student’st-tests (c–e); *P≤0.05, **P≤0.01, ***P≤0.05;n=10–15 mice per group. Figure 5: TrpC2 -mediated pheromone signals induce the loss of sexual olfactory preference and promote male-typical sexual behaviour. ( a ) Four-chamber social choice apparatus. Example of automated path tracking (curved line) of an experimental mouse, analysed with Ethovision software (Noldus). ( b ) Time spent (%) in each of the four chambers by laboratory and wild-backcrossed control and mutant TrpC2 females. ( c ) Number of females presenting male-typical mounting behaviour toward an alien male mouse. ( d ) Latency to first male-typical mounting behaviour toward alien adult male mice by laboratory and wild-backcrossed control and mutant females. ( e ) Duration of male-typical mounting attempts toward an alien adult male. Data are plotted as means±s.e.m., one-way analysis of variance followed by Fisher’s least significant difference post hoc test ( b ) or Student’s t -tests ( c – e ); * P ≤0.05, ** P ≤0.01, *** P ≤0.05; n =10–15 mice per group. Full size image A critical decision in animal-based research is to identify and select an appropriate animal model that enables in depth investigation of a specific biological phenomenon. By far, the most commonly used laboratory animal model for biological and biomedical studies is the laboratory mouse. The inbred laboratory mouse, with its thousands of inbred, specialized and genetically engineered strains, serves as a powerful tool for studying mechanisms underlying gene function in normal animal and human biology and in human diseases. An important feature of most laboratory mice is their relatively low genetic diversity and, as a consequence, their limited phenotypic variability. Although this selected and strain-specific phenotypic uniformity can be considered an advantage in empirical research, as the low heterogeneity of laboratory strains decreases phenotypic variability, thus necessitating fewer individuals in order to reach a significant conclusion, it also has certain disadvantages. More than three decades have passed since it was first reported that inbreeding and human selection for specific traits in typical laboratory mice lead to a loss or alteration of naturally occurring alleles and suppress natural behavioural traits (reviewed in ref. 30 ). It was therefore argued that domesticated inbred mice are, in many ways, poorly suited to serve as models of ‘normal’ mice. Furthermore, it was suggested that genetically modifiable strains derived from wild house mice might serve as useful models, especially for experimental work in behavioural and brain sciences [30] . Thus, findings obtained from studies in wild-derived stocks might provide valuable opportunities to unravel the relationships between genotype and complex natural phenotypic traits that are reduced or even absent in domesticated stocks [10] , [14] , for example agonist behaviours in males and females, resistance to capture by humans (reviewed in ref. 13 ), activity levels [31] and immune function [32] . In the present study, we showed that by simple classical backcrossing of wild mice with laboratory knockout models it is feasible to retain alleles lost during domestication and eliminate mutant alleles that accumulate in most typical laboratory stocks. Furthermore, to the best of our knowledge, this is the first demonstration of the powerful applicability of studies of wild-derived gene-targeted mouse models to provide new knowledge about ecologically relevant biological phenomena that up to now have been in typical models of domesticated laboratory mice. Surprisingly, our findings also demonstrated that the study of wild-backcrossed mice provides an opportunity to uncover novel behavioural gene functions in females, which are unique to ancestral wild mice and are absent in classical laboratory females. As an example, wild-derived females, but not laboratory females were found here to exhibit spontaneous freezing behaviour, aggression toward a same-sex alien adult mouse and aggression toward alien pups. In contrast, for most behavioural traits the differences between the male groups were only quantitative if they existed at all. The female bias in the effects of domestication on the behavioural phenotype may result from two processes. First, human selection pressure may have been higher on females than on males, and may have tended to eliminate females displaying inter-female aggression, intolerance to cage mates and aggressive behaviour toward newborn pups [33] . Alternatively or in addition, females may have adapted more rapidly and robustly to changes in social and environmental conditions in order to enhance successful breeding in the artificial laboratory conditions. Notably, in both sexes, two social behavioural measurements were expressed only in laboratory mice and not in wild or wild-backcrossed mice. This was in contrast to all other measured parameters, which were expressed at similar levels or more robustly in wild mouse strains. These phenotypic exceptions were same-sex mounting behaviour and pup-triggered parental behaviour in sexually naïve individuals, and may be the result of human positive selection favouring these traits to enhance breeding success under artificial laboratory conditions. With regard to the gene-expression profiles in the brain, as well as the phenotypes of both sexes, our wild-backcrossed mice were indistinguishable from the wild mice but differed greatly from the tested laboratory mice within the battery of assays performed. Importantly, wild-backcrossed females also manifested all behavioural traits that had been lost through domestication in laboratory females, including aggressive behaviour toward alien adults and newborn pups. These latter sets of behaviours are considered to be male-typical traits that are rarely exhibited by laboratory females [26] , [34] , [35] , [36] , whereas in nature they serve evolutionary adaptive purposes [26] , [37] and are robustly exhibited in both wild males and females, thus offering an unique opportunity for mechanistic investigation in both sexes. In the present study, we focused on assessing the role of TrpC2 in female conspecific aggressive behaviours. The behaviour characterization of wild-backcrossed TrpC2 -mutant demonstrates that aggressive behaviour towards pups and inter-female aggression in mouse models is largely regulated in both sexes by vomeronasal organ-mediated pheromone signals. This suggests that similar neuronal circuits, activated by common environmental sensory signals, might underlie and mediate this behaviour in both males and females [38] . These findings provide a foundation for future studies on the neuronal and molecular basis of ecologically relevant sexually dimorphic social and reproductive behaviours in females and are likely to contribute valuable new insights into the olfactory coding and evolutionary mechanisms underlying sex-specific pheromones. Studies on gene-targeted inbred laboratory mice have indeed provided the basis for a vast amount of our current biological knowledge. However, many gene-targeted mouse models are reported to possess no obvious behavioural phenotype, and as shown here, inbred mouse strains do not demonstrate the full range of the naturally occurring behavioural phenotype such as that exhibited by wild house mice. In this respect, wild-derived genetically targeted mouse models may serve as unique natural, evolutionarily relevant resources for many quantitative traits that might prove valuable in defining new gene—phenotype associations, leading to a better understanding of the genetic and neuronal bases of complex polygenetic traits. Given the extraordinary increase in targeted mouse model resources [4] and the availability of ‘speed congenic’ breeding methodology [23] , it will probably soon be possible to promptly generate, within four or five generations of breeding, a wild-backcrossed mutant mouse model for any gene in the mouse genome. Notably, during the backcrossing procedure, we observed (data not shown) that within three generations of backcrossing the wild-backcrossed mouse model exhibits behavioural traits strongly resembling those of the wild mice, including all the traits that were present in wild mice but absent in laboratory mice. This observation requires further study. Moreover, a novel technology (CRISPR-Cas9) was recently developed to allow generation of mutant mice by direct embryo manipulation [39] . Since this gene-targeted technology is not dependent on acquiring embryonic stem cells or on the genetic background of the genetically disrupted embryo, it can be directly applied to generate wild mutant mice for one or a few targeted genes. This would make it possible to dispense with the lengthy process of backcrossing, making the study of wild mutant mouse models more accessible and attractive. Such a procedure would open the way to initiating large-scale studies to re-evaluate the functions of genes for which no phenotype is observed in the classical laboratory mouse model, but may now be detectable in wild mutant models, thus providing a more physiological, ecologically relevant model system that should present richer and more complex behavioural traits. Another important potential application of wild-derived genetically modified mouse models is in preclinical and drug development studies. A major debate has recently emerged in the scientific community concerning the consistent neglect in the use of females as animal subjects in neuroscientific and biomedical studies related to mental disorders [40] , [41] , including sexually dimorphic disorders such as autism [42] and anxiety [43] . Gender biases in experimental cohorts have been reported to influence both the investigation of biological mechanisms underlying the diseases and the effectiveness of available drugs and treatments [40] , [41] , [44] . The present study demonstrated that in studies using typical domesticated laboratory mice, females more than males have been selected for enhancing docility and reduction in aggressive behaviour. The results of such phenotypic selection are likely to be associated with substantial alterations in key neurobiochemical (for example, serotonergic and dopaminergic [45] ) and neuroendocrine processes, and in the aetiology of many dimorphic neurodevelopmental disorders. Hence, the use of wild-derived female mice in biomedical and preclinical research may shed light on sex and gender factors affecting women’s health that cannot be achieved by studying only laboratory inbred females. To summarize, we suggest that a more comprehensive understanding of the complex genetic factors underpinning natural evolution-related social and reproductive behaviours, and new insights into the sexual dimorphism of brain functions in health and disease, can be obtained by the study of gene-targeted mutations in wild mutant strains. Moreover, natural polymorphic variant genes carried by wild-derived strains more closely resemble common human genetic variations than the genetic backgrounds of inbred mice, and these strains may thus better serve as models for understanding human complex biological systems such as the immune system [46] , as well as complex behaviours and polygenic complex diseases [9] , [47] , [48] . Thus wild-backcrossed mouse models should be seen as an important complementary tool, and possibly as a ‘missing link’ between laboratory-based mouse studies and genome-wide association studies in humans. Animals Sexually naive adult (14- to 18-week-old) mice from five different groups were used: (i) Laboratory mutant TrpC2 , (ii) laboratory control TrpC2 (note: in preliminary testing we found no significant differences between the TrpC2 +/+ and TrpC2 +/− genotypes; we therefore considered the heterozygous state as a valid control group), (iii) wild-backcrossed mutant TrpC2 , (iv) wild-backcrossed control TrpC2 and (v) wild ( TrpC2 +/+ ) mice. The genetic background of the laboratory TrpC2 mice was C57BL/6J × 129S1/Sv. Wild house mice were trapped in the fields (Idaho, USA) near livestock barns and kept under laboratory conditions for seven generations as an outbred stock of pathogen-free wild mice [20] . Wild-backcrossed mice were produced by 10-generation backcrossing of laboratory TrpC2 mice with wild house mice. To maintain high genetic and phenotypic diversity, we prevented inbreeding by not allowing crosses between siblings or between parents and offspring. All of the laboratory, wild and wild-backcrossed mice were raised and bred under the same standard pathogen-free laboratory conditions for several generations before being phenotypically characterized. Housing conditions Each strain was housed separately and in mixed genotype groups. Three or four mice were housed in a standard mouse cage (separated by sex). All mice were housed in the same mouse facility and received the same treatment. All were maintained on a 12 h/12 h light/dark cycle with food and water ad libitum . For 2 weeks before the start of behavioural assays, the mice were housed individually under a reverse light–dark cycle. At the time of all measurements, mice were adult and sexually naive (14–18 weeks old). All experimental procedures were approved by the Institutional Animal Care and Use Committee of The Weizmann Institute of Science. Physiological and morphological measurements Adult mice were individually housed in home cages with a measured quantity of food and water. After 6 days, any remaining food or water in the cages was weighed. Mice in each of the five groups were lightly anaesthetized and their body weight and length (excluding the tail) were measured. Body length was measured in accordance with the previously reported protocol: https://www.mousephenotype.org/impress/protocol/90/7 . Stress hormone measurements New groups of sexually naive adult mice were anaesthetized in the dark cycle (within 2−5 h into the beginning of the dark cycle), using isoflurane gas in their home cage and were then killed by decapitation. This procedure ensured minimum handling or other interference that might cause stress in the mice that might interfere with corticosterone level measurements; thus, we can assume that the measured levels are close to baseline. Blood was collected immediately postmortem and plasma was separated by centrifugation and stored at −80 °C until analysed. Basal corticosterone concentrations in the plasma were assayed by ELISA (Cayman Chemical) according to the manufacturer’s instructions. Behavioural assays Open-field test . Adult mice were transferred to the experiment room at least 2 h before the start of the experiment. The apparatus for behavioural testing consisted of a Plexiglas arena (50 × 50 × 44 cm) illuminated with a 120-lux bulb. The tested mouse was placed in the corner of the box and allowed to explore the arena freely for 10 min. Spontaneous jump attempts and freezing behaviour were quantified online using an automated video tracking system (VideoMot2; TSE Systems). Behaviour was also recorded using digital video cameras. Mean velocity and angular velocity were scored using EthoVision software (Noldus). Dark-light transfer test . The test apparatus was a rectangular Plexiglas box divided by a partition into a dark compartment (14 × 27 × 26 cm) and a 1050-lux illuminated light compartment (30 × 27 × 26 cm), connected by a small passage. Mice were transferred to the experiment room at least 2 h before the start of the experiment. They were placed in the dark compartment and allowed to explore the arena for 5 min. The total path travelled, latency to entering the light zone and the time spent in the centre of the arena were quantified online using an automated video tracking system (VideoMot2). Four-chamber olfactory choice test . Mice used as stimuli were adult females, adult males and 14-day-old C57BL/6 pups (Harlan Laboratories). Apparatus: experiments were carried out in a four-chamber rectangular plastic box (40 × 40 × 20 cm; see Fig. 5a ) with a central compartment providing free passage between the chambers. Experimental procedure: behavioural tests were conducted on three consecutive days. On day 1, the tested mouse was placed in the centre of the apparatus and allowed to explore the empty chambers freely for 5 min. On day 2, a transparent perforated plastic box (10 × 10 × 10 cm) was placed in the centre of each of the four chambers. A mouse was placed in the apparatus and allowed to explore it for 15 min. On day 3, the three stimulus animals were individually placed in one of the perforated plastic boxes, leaving an empty box in the last chamber. The tested mouse was then placed in the middle of the apparatus and allowed to explore for 5 min. The time spent in each chamber was recorded with EthoVision software. The side of the stimulus animals in the apparatus was counterbalanced. After each trial, the complete apparatus was cleaned with 70% ethanol. All tests were done during the dark period under a dim red light. Resident-intruder assay (adult-pup interactions) : Stimulus animals: three newborn pups (1−3 days old). Experimental procedure: the tested mouse was placed in the experiment room on the evening before the test. At the start of the trials, the three stimulus pups were placed in the corner of the home cage of the tested mouse (opposite the nest). The resident mouse was allowed to interact with the pups for 15 min. Behaviour was recorded using digital video cameras and was later scored using Observer XT software (Noldus). Scored behavioural parameters were aggressive attack, disregard of pups (no interaction), maternal behaviour (for example, retrieval behaviour, nesting, crouching, olfactory investigation). All tests were done during the dark period under a dim red light. Ethical considerations: all experiments were performed in accordance with IACUC guidelines governing research on animal behaviour. Taking into account the needs of the present study, care was taken to minimize any stress or suffering that might be imposed on animals. Pups that were attacked during the experiment were immediately removed from the cage and humanely euthanized. Resident-intruder assay (same-sex adult interactions) [15] . An alien mouse, matched for age, sex and strain, was introduced into the home cage of the tested adult mouse for 15 min. Behaviour was recorded using digital video cameras and later scored using Observer XT software (Noldus). Behavioural parameters included olfactory investigations, aggressive attacks and sexual mounting attempts. All tests were done during the dark period under a dim red light. Total RNA extraction and microarray assay Total RNA was extracted from the hypothalamus of wild mice and laboratory mice using a PerfectPure RNA Tissue Kit (5 Prime) according to the manufacturer’s protocol. RNA extracts were stored at −80 °C until use. For each condition, RNA from two mice (two arrays for each of the two mouse strains) was pooled, purified and hybridized to an Affymetrix GeneChip Mouse Gene 1.0 ST Array (Affymetrix, Santa Clara, CA). Labelling, hybridization and scanning of the microarray were performed at the Bioinformatics and Biological Computing Unit at the Weizmann Institute. Expression patterns were analysed using Partek Genomics Suite software (Partek, St Louis, MO). Affymetrix data were checked for possible differences in probe-binding affinity resulting from sequence differences between the laboratory strain and the wild strain using code based on the R-package maskBAD ( http://bioconductor.org/packages/2.10/bioc/html/maskBAD.html ). Only probe sets that were expressed in all eight samples were retained for the affinity test. None of the probes showed significant differences in binding between strains (false discovery rate, q >0.05 for all probes). RNA purification, cDNA synthesis and qPCR Total RNA from the hypothalamus of three adult mice of wild, wild-backcrossed and laboratory strains was extracted with TRI Reagent (Sigma-Aldrich) and purified using the RNeasy Kit (Qiagen). RNA was converted to cDNA using a High Capacity cDNA Reverse Transcription Kit (Applied Biosystems). The expression levels of specific mRNAs were assayed using Power SYBR Green PCR Master Mix (Applied Biosystems). Quantification reactions were performed in triplicate for each sample. Sequences of the primers used are recorded in Supplementary Table 2 . SNP array in wild-backcrossed TrpC2 mutant mice The flanking regions (proximal and distal) of the introduced TrpC2 -knockout locus were determined by genotyping of the entire (3.1−152.5 Mbp) chromosome 7 with 2,612 SNP markers using the MegaMUGA SNP array as described [22] and conducted by GeneSeek (Lincoln, NE, USA). The entire set of SNP markers was tested for 19 wild-backcrossed TrpC2 −/− and two inbred mouse strains (C57BL/6J and 129S1/Sv) and the F1 (C57BL/6J × 129S1/Sv Trpc2 −/− ) cross mice. These were designated as uninformative SNPs and therefore did not contribute to the analysis. Subsequently, all SNPs that had no calls in 95% of the inbred and F1 cross mice were filtered. These SNPs were also designated as uninformative markers. On the basis of mm9 (mouse map genome, July 2007) and the SNPs in dbSNP (build 128), the TrpC2 gene should reside at position chr7:109231630−109245378 (RefSeq). All SNP markers in the 19 wild-backcrossed TrpC2 −/− mice that were identical to those in the two inbred mouse strains and the F1 (C57BL/6J × 129S1/Sv Trpc2 −/− ) cross were marked in grey and are presented in Supplementary Data 1 . The largest SNP cluster around the TrpC2 gene that is shared between the F1 laboratory line and the 19 wild-backcrossed mice was between 106,614,708 and 114,745,432 bp, which spans approximately 8 Mbp. On the basis of this analysis, it was concluded that the introduced/congenic TrpC2 -knockout locus in the 19 wild mice was about 8 Mbp, and that both sides are flanked by wild genotypes. SNP array data have been deposited in the Gene Expression Omnibus. Statistical analyses All statistical analyses were performed using SPSS software (Chicago, IL, USA) and STATISTICA software (StatSoft, Tulsa, OK, USA). Results are presented as means±s.e.m. For comparisons between measurements of the different strains and genotypes, we used either Student’s t -test or one-way analysis of variance following post hoc Fisher least significant difference multiple comparison. * P ≤0.05, ** P ≤0.01, *** P ≤0.005. How to cite this article: Chalfin, L. et al . Mapping ecologically relevant social behaviours by gene knockout in wild mice. Nat. Commun. 5:4569 doi: 10.1038/ncomms5569 (2014).